Particle correlations and evidence for dark state condensation in a cold dipolar exciton fluid Dipolar excitons are long-lived quasi-particle excitations in semiconductor heterostructure that carry an electric dipole. Cold dipolar excitons are expected to have new quantum and classical multi-particle correlation regimes, as well as several collective phases, resulting from the intricate interplay between the many-body interactions and their quantum nature. Here we show experimental evidence of a few correlation regimes of a cold dipolar exciton fluid, created optically in a semiconductor bilayer heterostructure. In the higher temperature regime, the average interaction energy between the particles shows a surprising temperature dependence, which is evidence for correlations beyond the mean field model. At a lower temperature, there is a sharp increase in the interaction energy of optically active excitons, accompanied by a strong reduction in their apparent population. This is evidence for a sharp macroscopic transition to a dark state, as has been suggested theoretically. Different collective many-body effects in Bose quantum fluids of atoms [1] and exciton-polaritons [2] have been observed in recent years. The common feature of these quantum fluids is the weak interaction between the particles, which generally can be well described using mean field theories, where the interaction is considered as a local, contact-like scattering [1] . In contrast, cold dipolar fluids are composed of particles that carry a permanent electric dipole. Owing to the strength and longer range of the dipole–dipole interaction, dipolar fluids are predicted to display physics that goes beyond a mean field description [3] . In particular, cold dipolar bosons are expected to have new quantum as well as classical multi-particle correlation regimes [3] , [4] , [5] . Observing the many-body correlations will open a window to the complex underlying physics that may drive the fluid into different theoretically proposed collective phases such as dipolar superfluids, dipolar crystals and dipolar liquids [6] , [7] , [8] , [9] . There are currently only a few feasible realizations of quantum dipolar fluids that are being experimentally tested. Perhaps the most known are dipolar atoms [3] or polar molecules [10] in either magneto-optical traps or optical lattices [1] , and indirect dipolar excitons in semiconductor quantum structures [11] , [12] . Indirect dipolar excitons ( X id ) are coulomb-bound electron-hole pairs inside an electrically gated semiconductor bilayer (also known as a double quantum well (DQW)). X id are two-dimensional (2D) boson-like quasi-particles (see illustration in Fig. 1a ) with four quasi degenerate spin states (in GaAs based DQW structures). The two states with spin S =±1 are optically active (‘bright’) and the two states with spin S =±2 are optically inactive (‘dark’) [13] . The X id carry a static electric dipole because of the separation of the electron and the hole into the two adjacent layers. Furthermore, all the dipoles are aligned perpendicular to the layers, so that the dominant interaction between the X id is an extended repulsive dipole–dipole interaction [14] , [15] . The unique advantage of X id systems is that the effect of the interactions between the excitons can be observed directly: the interaction of a given exciton with its surrounding excitons is manifested in an excess energy (called the ‘blue shift’ −Δ E ), carried away from the system by a photon as the exciton recombines radiatively. It was suggested theoretically that this observed interaction energy could be used as a direct experimental probe of the various particle correlation regimes and the thermodynamic phases of X id systems [5] , [15] , if it can be mapped as a function of the fluid temperature and density [16] , [17] . However, calibrating the fluid density reliably at different temperatures turned out to be a non-trivial task in optically excited exciton systems [18] , which so far hindered direct and consistent observations of interaction-induced particle correlations. On the other hand, recent works have shown other manifestations of a spontaneous transition to a macroscopic condensed state of X id , such as an extended optical coherence of the X id emission [12] , [19] , [20] , as well as persistent spin textures [12] in excitonic rings [21] , [22] . 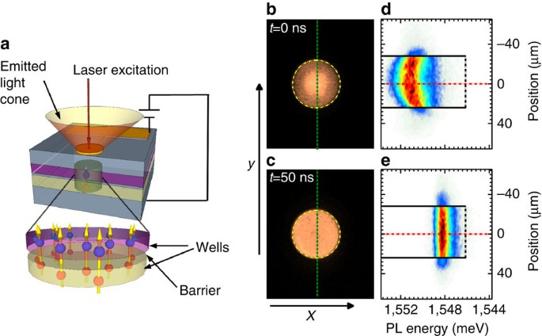Figure 1: Dipolar excitons in an electrostatic trap. (a) An illustration of the bilayer system, the dipolar excitons and the circular electrostatic trap gate geometry. The excitation laser pulse impinges at the centre of the trap. (b–e) PL of anXidfluid inside an electrostatic trap at two different times after a non-resonant excitation pulse. The first stage of the dynamics starts with a fast expansion of the dense and hot carriers due to the carrier–carrier repulsion (not seen here), followed by a cooling and a formation of Xid. Owing to their strong dipole–dipole repulsion, theseXidcontinue to expand rapidly towards the edges of the circular trap26, where they are confined through the interaction of their dipole with the externally applied electric field under the trapping gate. (b,c) Real space images of theXidfluid PL from an electrostatic trap (b) during the laser pulse and (c) 50 ns after the laser pulse. The PL is spectrally filtered to collect only the emission from theXidfluid. Note that theXidfluid reaches a homogeneous distribution in the trap inc. The dashed yellow line mark the trap's gate boundary. (d,e) Spectral colormap images (in log scale) of theXidPL, taken from the cross-sections of the electrostatic trap, shown by the green dash lines inb,c. The dot-dashed red line marks the spatial location of the excitation spot and the horizontal black lines mark the trap’s gate boundary. The vertical black dot-dashed line marks the energy at the bottom of the trap. The PL is clearly blue shifted with respect to this energy due to mutual dipolar interactions between particles. Figure 1: Dipolar excitons in an electrostatic trap. ( a ) An illustration of the bilayer system, the dipolar excitons and the circular electrostatic trap gate geometry. The excitation laser pulse impinges at the centre of the trap. ( b – e ) PL of an X id fluid inside an electrostatic trap at two different times after a non-resonant excitation pulse. The first stage of the dynamics starts with a fast expansion of the dense and hot carriers due to the carrier–carrier repulsion (not seen here), followed by a cooling and a formation of X id . Owing to their strong dipole–dipole repulsion, these X id continue to expand rapidly towards the edges of the circular trap [26] , where they are confined through the interaction of their dipole with the externally applied electric field under the trapping gate. ( b , c ) Real space images of the X id fluid PL from an electrostatic trap ( b ) during the laser pulse and ( c ) 50 ns after the laser pulse. The PL is spectrally filtered to collect only the emission from the X id fluid. Note that the X id fluid reaches a homogeneous distribution in the trap in c . The dashed yellow line mark the trap's gate boundary. ( d , e ) Spectral colormap images (in log scale) of the X id PL, taken from the cross-sections of the electrostatic trap, shown by the green dash lines in b , c . The dot-dashed red line marks the spatial location of the excitation spot and the horizontal black lines mark the trap’s gate boundary. The vertical black dot-dashed line marks the energy at the bottom of the trap. The PL is clearly blue shifted with respect to this energy due to mutual dipolar interactions between particles. Full size image In this paper, we show experimental evidence of a few correlation regimes of a cold dipolar exciton fluid, created optically in a semiconductor bilayer heterostructure. In the higher temperature regime, the average interaction energy between the particles shows a temperature dependence that is an evidence for correlations beyond the mean field model. At a lower temperature, there is a sharp increase in the interaction energy of optically active excitons, which is accompanied by a strong reduction in their apparent population. This could be an evidence for a sharp macroscopic transition, where the fluid redistribute its density with dark states that are uncoupled to light, as was suggested theoretically [13] . Experimental scheme Here we present time-resolved photoluminescence (PL) experiments of an optically excited X id fluid trapped inside an electrostatic trap [23] , [24] , [25] , [26] . We extract a consistent mapping of Δ E for a range of bright exciton densities ( n b ) and temperatures. Figure 1b,c show typical time-resolved PL images of an X id fluid inside an electrostatic trap after its excitation with a non-resonant-pulsed laser. About 50 ns after excitation, the fluid reaches a dynamic equilibrium between the dipole–dipole repulsion of excitons that tends to drive the fluid outwards, and the confining ‘flat well’ potential induced by the electrostatic gate [27] . This equilibrium results in a uniform and homogeneous PL distribution inside the trap, indicating a flat density profile. This is clearly seen in Fig. 1c,d,e present the corresponding spatial-spectral images taken along the central axis of the trap gate. Figure 1e shows that the homogeneously distributed PL is blue shifted from the emission energy of a single exciton. This positive blue shift energy Δ E id is due to the repulsive dipole–dipole interaction inside the X id fluid. In general, Δ E increases as n b increases and its value is sensitive to the intricate multi-particle correlation [5] , [15] . 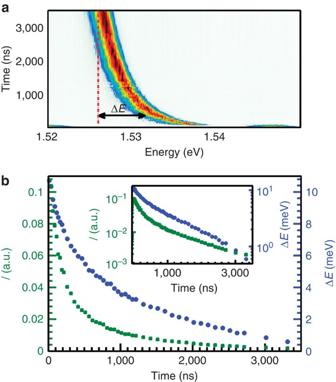Figure 2: PL dynamics of a trappedXidfluid. (a) Spatially integrated PL spectra of anXidfluid in a trap (taken at 3K) at different times after the short excitation pulse. The intensities are all normalized to unity for convenience. The dot-dashed red line indicates the extrapolatedXidenergy as the density of the bright excitons goes to zero. The blue shift energy, ΔE, is measured from this extrapolated energy as is marked by the black arrow. (b) The extracted time dependence ΔE(blue circles) and the integrated intensityI(green squares) from theXidspectra ina. It is seen that ΔEandIdecay non-exponentially and at different rates because of the dependence of the effectiveXidlifetime on ΔE(see text). The inset presents the same data as inbbut in log scale. Analysis of the X id lifetime Figure 2a presents an example of the spatially integrated and normalized PL spectra, taken at T =3 K at different times after the excitation pulse. The spectral position of the PL line shifts with time to lower energies as n b decreases. At long times, the PL energy asymptotically reaches a constant value. The difference between the PL energy at any given time to this asymptotic value is the blue shift energy Δ E (marked by the arrow in Fig. 2a ). The time dependence of the spectrally integrated PL intensity ( I ) and Δ E are plotted in Fig. 2b . As the X id density drops with time, both I and Δ E decreases with a non-exponential decay rate. The reason for this non-exponential decay is the dependence of the X id radiative recombination time ( τ id ) on n b : as is illustrated in Fig. 3a , radiative recombination of the X id can be described by a tunelling of either the electron or the hole (with a much lower probability because of its larger mass) to the adjacent well, where direct optical recombination with the oppositely charged particle takes place with a direct exciton recombination time τ d . The tunnelling probability depends on the difference between the direct and indirect transition energies, E d − E id . The larger the energy difference, the larger the τ id compared with τ d . This picture can be quantified to get an expression for τ id in terms of τ d and E d − E id (see Supplementary Note 1 ): Figure 2: PL dynamics of a trapped X id fluid. ( a ) Spatially integrated PL spectra of an X id fluid in a trap (taken at 3 K ) at different times after the short excitation pulse. The intensities are all normalized to unity for convenience. The dot-dashed red line indicates the extrapolated X id energy as the density of the bright excitons goes to zero. The blue shift energy, Δ E , is measured from this extrapolated energy as is marked by the black arrow. ( b ) The extracted time dependence Δ E (blue circles) and the integrated intensity I (green squares) from the X id spectra in a . It is seen that Δ E and I decay non-exponentially and at different rates because of the dependence of the effective X id lifetime on Δ E (see text). The inset presents the same data as in b but in log scale. 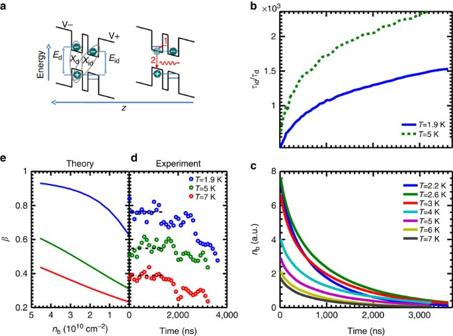Figure 3: Density calibration and thermal distribution of theXidfluid. (a) On the left side, a schematic illustration of the energy band diagram of a DQW (in the growth direction) under an applied bias is shown . The energies of the direct exciton (Ed) and the dipolar exciton (Eid) are marked. The right side illustrates the process of anXidoptical recombination in which the electron effectively tunnels to the adjacent well (stage 1) and recombines with the hole (stage 2), emitting a photon. (b) Extractedτid/τdversus time for two experimental temperaturesT=1.9 and 5K, using equation (1). (c) The bright exciton density,nb(t), as a function of time for different temperatures, extracted using the calibration procedure described in the text. (d) The experimentally obtained values ofβat different times for three different temperatures. (e) Calculated values ofβas a function ofnbfor the same temperatures as indusing an ideal 2D BE thermal distribution. Full size image Figure 3: Density calibration and thermal distribution of the X id fluid. ( a ) On the left side, a schematic illustration of the energy band diagram of a DQW (in the growth direction) under an applied bias is shown . The energies of the direct exciton ( E d ) and the dipolar exciton ( E id ) are marked. The right side illustrates the process of an X id optical recombination in which the electron effectively tunnels to the adjacent well (stage 1) and recombines with the hole (stage 2), emitting a photon. ( b ) Extracted τ id / τ d versus time for two experimental temperatures T =1.9 and 5 K , using equation (1). ( c ) The bright exciton density, n b ( t ), as a function of time for different temperatures, extracted using the calibration procedure described in the text. ( d ) The experimentally obtained values of β at different times for three different temperatures. ( e ) Calculated values of β as a function of n b for the same temperatures as in d using an ideal 2D BE thermal distribution. Full size image where is the probability for an electron to tunnel to the hole QW, and v is the tunnelling matrix element. Note that although the non-polar, direct transition energy E d is independent of density, the dipolar energy E id depends on n b . The time dependence of τ id / τ d can be extracted from equation (1) by plugging in it the experimental values of E d − E id ( t ). Figure 3b presents this time dependence for the two exemplary temperatures of 1.9 and 5 K . Density calibration and thermal distribution of the X id fluid Because the dominant X id recombination channel is radiative [21] , [22] , [28] , the dynamics, and its relation to the observed PL intensity, can be described by a simple rate equation. Assuming an equilibrium of bright and dark X id with equal densities [29] (that is, n b =n d , where n d is the dark X id density), we get: where n rad is the density of optically active excitons with in-plane k -vectors that are inside the radiation light cone, β≡ ( n rad / n b ), and α ( T ) is the fraction of the total emitted photon flux that is collected by the detector (see Piermarocchi et al. [30] and Supplementary Note 2 for more information). We now note that counting all the emitted photons from a given time t after the excitation to t →∞ (where n b =0 ) yields n b (t) , that is, Combining equation (2) with equation (3), we get a relation between I ( t ), τ id ( t ) and β ( T ): As τ id was extracted independently from the PL energy using equation (1), comparing the two sides of the equation yields β (T,t) . This dependence is plotted for three different temperatures in Fig. 3d . β increases with decreasing time, that is, with increasing n b . Also, β decreases with temperature. This density dependence is a signature of a deviation from a pure classical ideal gas distribution. Figure 3e plots the theoretically calculated values of β ( n b ) for the three corresponding temperatures using an ideal 2D Bose–Einstein (BE) model (see Supplementary Note 2 for the full derivation). There is a reasonable qualitative agreement between the calculation and the experiment, indicating the validity of the model assumptions. However, it is noteworthy that currently we cannot obtain a direct comparison between the theoretical and experimental values of β , as no absolute measurement of n b exists. Another strong verification for the validity of the above analysis was done for a trapped X id fluid in a steady state under a non-resonant continuous wave laser excitation and is shown in Supplementary Note 3 . 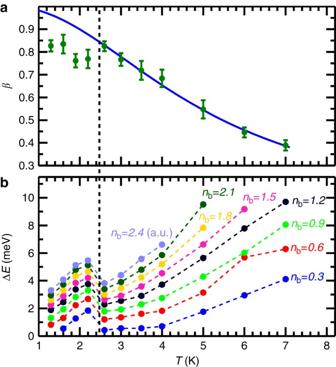Figure 4: Particle correlation regimes of anXidfluid. (a)βvalues at the high exciton density limit (marked by the black dashed lines inFig. 3d), as a function ofT(green circles), the error bars are calculated from the data inFig. 3d. The solid blue line is the theoretical values ofβ, assuming an ideal 2D BE thermal distribution withnb=3.5 × 1010cm−2. (b) ΔEas a function ofTfor different values of bright exciton densities,nb(dashed lines are guides to the eye). The vertical black dashed line markTc, the boundary between the two regimes as is discussed in the text. A lower bound fornbcan be obtained from the blue shift at the highest temperature by applying the mean field model5, yieldingnb≥2.2 × 1010cm−2/1 (a.u.). For this density estimate ,we assume that at the highest temperature, the bright and dark exciton densities are identical, and thereforenbis half of the total particle density. Evidence for correlations in the X id fluid Figure 4a shows in green circles the temperature dependence of β at the high-density limit (marked by the black dashed lines in Fig. 3d ). β ( T ) increases as T decreases down to ~2.5 K, where it suddenly drops. This behaviour is fitted to an ideal BE distribution, shown by the solid blue line. For temperatures above ~2.5 K, the theoretical prediction fits well with the experimental data. This means that for T 2.5 K, the X id fluid has a well-defined thermal distribution, but sharply deviates from it at lower temperatures. This is the first important observation of this analysis. Figure 4: Particle correlation regimes of an X id fluid. ( a ) β values at the high exciton density limit (marked by the black dashed lines in Fig. 3d ), as a function of T (green circles), the error bars are calculated from the data in Fig. 3d . The solid blue line is the theoretical values of β , assuming an ideal 2D BE thermal distribution with n b =3.5 × 10 10 cm −2 . ( b ) Δ E as a function of T for different values of bright exciton densities, n b (dashed lines are guides to the eye). The vertical black dashed line mark T c , the boundary between the two regimes as is discussed in the text. A lower bound for n b can be obtained from the blue shift at the highest temperature by applying the mean field model [5] , yielding n b ≥2.2 × 10 10 cm −2 /1 (a.u.). For this density estimate ,we assume that at the highest temperature, the bright and dark exciton densities are identical, and therefore n b is half of the total particle density. Full size image Next, we would like to map the dependence of Δ E on T and n b . This can be done with a common experimental calibration for the optically active exciton densities for all temperatures using equation (3). To do this in a simple tractable manner, we calculate an approximate, density independent value of α ( T ). We can then use this calculated value with equation (3) and the experimental values of I ( t ) to get n b ( t ) for each T . The results are plotted in Fig. 3c . This procedure allows us to compare the behaviour of the X id fluid with similar densities but at different temperatures. Figure 4b presents the experimental dependence of Δ E on T for different fixed densities. Two distinct temperature regimes are observed for all densities, corresponding exactly to the two regimes seen for β ( T ), with a sharp transition between them at T c 2.5 K. For all temperatures above T c , a clear temperature dependence of Δ E is observed. Δ E decreases with decreasing T . This dependence is a clear evidence for particle correlations beyond mean field. In contrast, a mean field calculation of Δ E predicts a ‘capacitor formula’ dependence that is temperature independent [31] . As the dipole–dipole interaction between the excitons is repulsive, a reduction of Δ E for a given density n b means an increase in the particle correlations: the more the X id spatially correlate to minimize their energy, the smaller Δ E will be. Therefore, the results suggest that as T decreases, the spatial correlations of the excitons in the fluid increase. To better quantify the dependence of Δ E and therefore the particle correlations on n b and T in this regime, we look for a scaling law of our data. 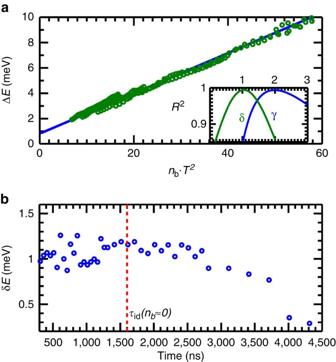Figure 5: Analysis of the dipolar interaction energy. (a) Scaling of the data of ΔEinFig. 4btonbT2for allT>Tc. The solid straight line was added as a guide to the eye. The inset shows theR2values of the quality of scaling of the experimental ΔEdata tonbδTγfor different values of the exponentsγandδ. (b) The time dependence of the magnitude of the energy ‘jump’ given byδE=Eid(T=2.2K)−Eid(T=2.6K), where these two temperatures correspond to the temperatures just below and aboveTc, respectively. The dashed red line marks the value ofτid(T=2.2K) at the low density limit. Figure 5a plots Δ E for a large set of densities and for all the measured temperatures above, as a function of n b T 2 . The data collapse into a single linear line to a high accuracy (see inset). The linear dependence of Δ E on n b suggests a lack of long range order in the fluid [5] . The scaling of Δ E on T 2 is surprising. In contrast, the models of Laikhtman and Rapaport, and Schindler and Zimmermann [15] predict a much weaker, sublinear dependence of Δ E on T , if the dipoles are a classically correlated gas. This specific temperature dependence could be an indication for a transition of the fluid correlations from classical to quantum. Although the former are expected to lead to a clear temperature dependence of Δ E , the latter should have a much weaker dependence, as was calculated in Laikhtman and Rapaport [5] . This transition to a temperature independent Δ E is especially clear for the low densities of Fig. 4b , and it happens at a temperature range very similar to the one where quantum degeneracy of X id was reported very recently [12] . Lower bound estimation for the X id density (see caption of Fig. 4b ) indeed suggests that the X id fluid should become quantum degenerate (see Supplementary Fig. S3 ) for all the densities presented. Figure 5: Analysis of the dipolar interaction energy. ( a ) Scaling of the data of Δ E in Fig. 4b to n b T 2 for all T>T c . The solid straight line was added as a guide to the eye. The inset shows the R 2 values of the quality of scaling of the experimental Δ E data to n b δ T γ for different values of the exponents γ and δ . ( b ) The time dependence of the magnitude of the energy ‘jump’ given by δE = E id ( T =2.2 K )− E id ( T =2.6 K ), where these two temperatures correspond to the temperatures just below and above T c , respectively. The dashed red line marks the value of τ id (T=2.2 K ) at the low density limit. Full size image Evidence for X id density redistribution in dark states Turning to the other regime, we observe a sharp increase in Δ E for all densities just below T c . This jump correlates well with the onset of the deviation from the theoretical values of β plotted in Fig. 4a , where we observe a sharp drop of β ( T < T c ) with much less radiative X id than the theoretical prediction of a BE gas of bright excitons (plotted in blue). In other words, suddenly below T c , there seem to be less bright excitons but yet more interaction energy. This could be an indication for a sudden and sharp depletion of the bright exciton density and a sudden macroscopic transition to an optically inactive ‘dark’ state below T c . This increase in the density of the dark state can be seen in Δ E of bright excitons, as these dark excitons still interact with the bright excitons. A BE condensation (BEC) of dark excitons and its effect on the excited bright exciton energy was recently suggested in a theoretical paper by Combescot et al. [13] It was proposed that in perfect excitonic systems, the dark excitons should have an energy slightly lower than the bright excitons, and therefore at low enough temperatures and high densities, a BEC should form in the dark state. The following possible scenario is therefore consistent with our experimental observations: for all temperatures, the pulse excitation creates a large density of hot particles that very quickly (within a few nanoseconds) cool down to the lattice temperature. For T > T c , due to efficient spin flip processes between dark and bright states [29] , [32] , their population is approximately equal throughout the optical recombination process and their density decay together with time (that is, n b ( t )= n d ( t ) for all t ). At temperatures below T c , the high-density fluid cools down and condenses fast after excitation, pulling bright excitons to the dark ground state so that the population equality between the two species breaks down, resulting in more dark excitons and less bright excitons than expected ( n b < n d ), as is seen in Fig. 4a,b . The fact that the temperature dependence of this transition is very sharp (a fraction of a Kelvin), excludes the possibility of a simple thermal re-population of a lower dark state, but rather indicates to a sharp macroscopic transition. With the above picture in mind, it is expected that after the condensation, the scattering between the condensed particles in the fluid will be strongly suppressed, leading to a suppression of spin flip processes and therefore to an effective decoupling of the dark X id from the bright ones. An evidence for spin-scattering suppression was recently observed and analysed theoretically [12] . As the condensation and the bright–dark decoupling happens shortly after the pulsed excitation, it should be hard to directly observe the existence of a dark state by monitoring the dynamics of the bright X id PL intensity alone. However, there is a way to probe the dark state existence, as can be seen from Fig. 5b . Here we plot the time dependence of the energy ‘jump’ given by δE(t) = E id ( t , T =2.2 K )− E id ( t , T =2.6 K ), where these two temperatures correspond to the temperatures just below and above T c respectively. It can be seen that δE persists for times much longer than even the longest bright exciton lifetime (marked by the red dashed line), which indicates that there is a dark long-lived state in the system affecting the energy of the bright X id via mutual dipolar interactions. This observation is consistent with a dark excitonic state. A darkening of the PL of X id in a centre of stress-induced trap was recently observed by Sinclair et al. [33] In that work, the observed darkening was successfully explained by a position-dependent mixing of light- and heavy-hole X id , which have different emission rates. This mixing was induced by the inhomogeneous strain along the trap cross-section, and is essentially a single-particle effect, in contrast to a collective many-body effect. Their explanation could not, however, account for the temperature-dependent onset of their observed darkening. Therefore, it was suggested in Sinclair et al. [33] that perhaps many-body effects, and in particular dark–bright exciton splitting and dark exciton BEC, could be also involved; however, these effects could not be isolated. As the same strain fields are also expected to mix bright and dark excitons, it further complicates the interpretation. In our experiments, the trap is electrostatic, with a flat homogeneous electric field distribution all across the trap profile (except at the trap edges), so such mixing of light- and heavy-hole X id is not seen or expected, yet a significant darkening is observed. Furthermore, here we have a separate account of Δ E , which is proportional to the total X id density ( n b + n d ), and of n b alone. This allows us to separate the two types of states and to show that it is really a sharp reduction of emitting particle density and not of the total particle density that occurs across T c . We are also able to show that the two populations have very different lifetimes, as is expected from a decoupled bright and dark states. It may well be that some of the underlying physics responsible for the observations in Sinclair et al. [33] and in the present work are similar. This is an exciting and interesting possibility; however, a direct comparison between the two experiments should be taken with care. Finally, it may seem from Fig. 4b that T c is independent of particle density, but this might be misleading: note that in this figure, the different Δ E ( T ) curves are plotted for fixed n b rather than for the total X id density. In this plot, for every temperature, the different points of Δ E, which correspond to different n b 's, all come from the same experiment (different times after the pulse excitation). As for all T 's the initial excitation was the same, it is reasonable that the initial total particle densities were approximately the same. As T c is expected to depend on the total density right after thermalization (that is, at short times after the excitation), T c should be fixed by this experimental condition. Therefore, the persistent energy ‘jump’ δE for many values of n b reflects the very long lifetime of the effect, as was explained above. To summarize, the above results show a few distinct correlation regimes of a 2D dipolar exciton fluid. We note that because of the complexity of the system and the inherent problems of measuring a dark state directly, a consistent theoretical framework that can describe these effects, as well as further experimental efforts, are therefore an outstanding challenge. Sample The sample that is used in the experiment is a bilayer structure consisting of a 120/40/120Å—GaAs/Al 0.45 Ga 0.55 As/GaAs DQW on top of a n-doped GaAs substrate grown by molecular beam epitaxy. The bilayer structure consists, which serves as a bottom electrode. A semi-transparent metallic Ti circular electric gate, with a 50-μm diameter, is micro-fabricated on top of the structure and is connected to a top electrode, as illustrated in Fig. 1a . The area of the circular gate forms an electrostatic trap for the X id [34] , which remain confined under it. The DQW structure is placed much closer to the bottom electrode than to the top gates in order to prevent a significant charge separation that can occur on the boundary of the trap [23] , [24] , [35] . Experimental setup The sample is mounted into a liquid 4 He optical cryostat (Janis). The sample temperature in these experiments was varied in the range of 1.3–7 K. The sample is excited non-resonantly with a 671-nm Q-switched laser with a pulse duration of 15 ns and a repetition rate of 25 kHz, focused on the centre of the trap gate. The time and spatially resolved spectral images following the excitation pulses are collected by a fast-gated intensified CCD camera (PIMAX-II) mounted on a spectrometer (Princeton Instruments). How to cite this article: Shilo, Y. et al. Particle correlations and evidence for dark state condensation in a cold dipolar exciton fluid. Nat. Commun. 4:2335 doi: 10.1038/ncomms3335 (2013).